Origin of slow magnetic relaxation in Kramers ions with non-uniaxial anisotropy Transition metal ions with long-lived spin states represent minimum size magnetic bits. Magnetic memory has often been associated with the combination of high spin and strong uniaxial magnetic anisotropy. Yet, slow magnetic relaxation has also been observed in some Kramers ions with dominant easy-plane magnetic anisotropy, albeit only under an external magnetic field. Here we study the spin dynamics of cobalt(II) ions in a model molecular complex. We show, by means of quantitative first-principles calculations, that the slow relaxation in this and other similar systems is a general consequence of time-reversal symmetry that hinders direct spin–phonon processes regardless of the sign of the magnetic anisotropy. Its magnetic field dependence is a subtle manifestation of electronuclear spin entanglement, which opens relaxation channels that would otherwise be forbidden but, at the same time, masks the relaxation phenomenon at zero field. These results provide a promising strategy to synthesize atom-size magnetic memories. The discovery [1] of magnetic hysteresis near liquid helium temperatures in high-spin molecular clusters, such as Mn 12 acetate, made these molecules promising candidates to act as either magnetic memories or quantum bits. However, fulfilling this promise, that is, synthesizing molecules with magnetic memory above room temperature has proven to be a hard nut to crack. In close analogy with conventional magnetic bits, the slow relaxation of these single-molecule magnets (SMMs) arises from their strong magnetic anisotropy [2] , [3] . The spin reversal is hindered by the presence of energy barriers separating states with opposite spin orientations M s along the anisotropy axis. In the simplest case of easy-axis uniaxial anisotropy, the barrier height amounts to approximately | D | S 2 , where D <0 is a second-order axial anisotropy parameter and S is the molecular spin. Main efforts in this field have therefore been directed towards enhancing either D or S , or both. The negative sign of D (easy axis) was considered to be an important requirement because it energetically favours high | m S | states. If, by contrast, D is positive (easy plane) the ground state will be the m S =0 singlet for systems with integer S and the m S =±1/2 Kramers doublet for those with half-odd S . In a classical picture, a system with D >0 has no barrier, as the spin is free to rotate within the easy plane, unless there is some in-plane anisotropy, for example, given by a E ( S x 2 − S y 2 ) term, where E is a second-order rhombic anisotropy parameter. Even then, the barrier height is expected to be significantly reduced with respect to the easy-axis case because of the condition | E |≤ D /3, and spin tunnelling rates are expected to be much higher, both of which contribute to erase magnetic memory. In 2012, Long and colleagues [4] found that a mononuclear pseudo-tetrahedral Co II complex, [Co II (Cl)L] + (L: 1,1,1-tris-[2 N -(1,1,3,3-tetramethylguanidino) methyl]ethane) with D >0 shows slow magnetic relaxation, that is, it behaves as an SMM, when a small static magnetic field is applied to it. The same or similar behaviour has thereafter been reported for a number of other Co II complexes [5] , [6] , [7] , [8] , [9] as well as for lineal Fe II complexes [10] . However, a detailed microscopic interpretation of this phenomenon is still missing. In some cases [5] the temperature dependence of the spin–lattice relaxation rate could be fitted using the exponential dependence expected for a thermally activated, or Orbach [11] , process, with activation energies U that are not far from the classical energy barrier ES 2 associated with the in-plane anisotropy. However, this interpretation is incompatible with the energy level schemes of Co II complexes, which consist of only two Kramers doublets separated by an energy gap Δ >> ES 2 and with the fact that Orbach processes imply phonon-induced transitions to ‘real’ intermediate spin states [11] . The goal of the present work is to perform a complete study of a Co II model complex [12] , [13] , [14] , [Co(acac) 2 (H 2 O) 2 ] (acac=acetylacetonate) hereafter referred to as complex ( 1 ), which has a very large positive D (≈57 cm −1 ), and to propose a new mechanism to consistently explain the spin–lattice relaxation of such systems. The results show that slow magnetic relaxation ensues naturally from Kramers theorem, irrespective of the sign of D , and that the magnetic field dependence of the linear dynamical response reflects the existence of a strong electronuclear spin entanglement. Magnetic anisotropy and spin Hamiltonian The molecular structure of ( 1 ) is shown in Fig. 1 . Each Co II ion occupies a site with distorted octahedral symmetry. The interaction with the crystal field stabilizes an orbital singlet with a high spin S =3/2 and a sizeable zero-field splitting. The electronic spin is subject to the action of external magnetic fields and to the hyperfine interaction with the I =7/2 nuclear spin of Co. 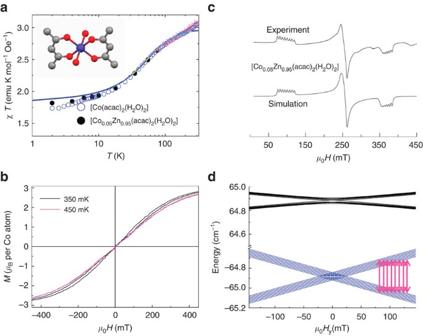Figure 1: Magnetic properties and anisotropy. (a) Temperature dependence of the product of the magnetic susceptibilityχtimes the temperatureTfor pure (open symbols) and magnetically diluted (solid symbols) samples of (1). Magenta stars are data from ref.14. The solid line is a theoretical prediction that follows from equation (1). TheχTdrop observed below 5 K for the pure sample is associated with intermolecular magnetic interactions, which are suppressed upon diluting CoIIwith diamagnetic ZnII. The inset shows the molecular structure of (1). (b) Magnetization hysteresis curves measured at different temperatures on a single crystal of (1) by sweeping the magnetic field along itsbcrystallographic axis at a rate of 12.6 mT s−1. (c) X-band EPR powder spectrum of the diluted sample, compared with a simulation based on equation (1). (d) Magnetic energy levels of theS=3/2 ground multiplet calculated using the spin Hamiltonian (equation (1)) with a magnetic field applied along the easy axisy(notice the broken energy axis). Below 30 K, the population of the ground electronic doublet exceeds 0.999, thus the system behaves as an effective electronic spin 1/2 system, split by Zeeman and hyperfine interactions. Magenta arrows show EPR transitions between states with the same nuclear spin state (ΔmI=0). The magnetic behaviour of ( 1 ) can be approximately described with the following effective spin Hamiltonian Figure 1: Magnetic properties and anisotropy. ( a ) Temperature dependence of the product of the magnetic susceptibility χ times the temperature T for pure (open symbols) and magnetically diluted (solid symbols) samples of ( 1 ). Magenta stars are data from ref. 14 . The solid line is a theoretical prediction that follows from equation (1). The χT drop observed below 5 K for the pure sample is associated with intermolecular magnetic interactions, which are suppressed upon diluting Co II with diamagnetic Zn II . The inset shows the molecular structure of ( 1 ). ( b ) Magnetization hysteresis curves measured at different temperatures on a single crystal of ( 1 ) by sweeping the magnetic field along its b crystallographic axis at a rate of 12.6 mT s −1 . ( c ) X-band EPR powder spectrum of the diluted sample, compared with a simulation based on equation (1). ( d ) Magnetic energy levels of the S =3/2 ground multiplet calculated using the spin Hamiltonian (equation (1)) with a magnetic field applied along the easy axis y (notice the broken energy axis). Below 30 K, the population of the ground electronic doublet exceeds 0.999, thus the system behaves as an effective electronic spin 1/2 system, split by Zeeman and hyperfine interactions. Magenta arrows show EPR transitions between states with the same nuclear spin state ( Δm I =0). Full size image where ĝ and Â hf are the gyromagnetic and hyperfine tensors, respectively. The nuclear quadrupole term is omitted, as its effect is not detectable in the electron paramagnetic resonance (EPR) spectra. Molecular orbital calculations, described in Supplementary Note 1 , and crystal-field arguments [15] suggest that the slightly distorted octahedral coordination of Co II cations, showing elongated Co–O bonds with the water molecules in comparison with those corresponding to the acac ligands, favours an easy-plane magnetic anisotropy. This qualitative analysis has been corroborated by ab initio calculations, performed using CASSCF and CASPT2 methods adding spin–orbit effects with the RASSI method. The results (see Table 1 ) give a positive D value together with a relative large E . The inclusion of dynamic correlation with the CASPT2 method gives rise to a smaller spin–orbit effect resulting in smaller anisotropy parameters. The splitting between the two Kramers doublets remains nevertheless larger than 130 cm −1 (see Table 1 ), a value that is within the characteristic range observed for other hexacoordinate Co II complexes [5] , [16] . The sign of D agrees also with that predicted by previous DFT calculations [17] , although the latter predict a weaker magnetic anisotropy. Table 1 Results of ab initio calculations. Full size table The parameters of equation (1) have been refined by fitting equilibrium magnetic susceptibility χ data and low temperature EPR spectra, shown in Fig. 1 . The temperature dependence of the χ T product is fully compatible with the sign and intensity (namely with D ≈57 cm −1 ) of the anisotropy derived from ab initio calculations, thus confirming that the zero-field splitting is of order 130 cm −1 . The analysis of EPR data, described in Supplementary Note 2 , provides further information on the nature of the electronic ground state doublet and the magnetic anisotropy terms. These results, summarized in Supplementary Fig. 1 and Supplementary Table 1 , reveal the presence of a strong in-plane anisotropy and a ratio E / D =0.31, larger than that predicted by ab initio calculations. The fit also requires introducing a slight anisotropy in the gyromagnetic tensor of equation (1), with principal values g x =2.50, g y =2.57 and g z =2.40. The principal values of the hyperfine tensor A xx =19(1) × 10 −4 cm −1 , A yy =76(1) × 10 −4 cm −1 and A zz =48(1) × 10 −4 cm −1 agree with those reported by Bencini et al [12] . Equation (1) also accounts very well for the equilibrium magnetization and magnetic heat capacity of ( 1 ) measured at different temperatures and magnetic fields, as shown by Supplementary Figs 2, 3 and 4 . Experimental study of spin–lattice relaxation The spin–lattice relaxation has been studied by means of frequency-dependent ac susceptibility experiments performed on magnetically diluted samples [Co x Zn 1− x (acac) 2 (H 2 O) 2 ], with x =0.05, complex ( 2 ). This reduces the strength of intermolecular magnetic interactions, which, as shown by Supplementary Fig. 5 , strongly influence the spin dynamics in concentrated samples. Representative data, measured at 1.8 K under different magnetic fields, are shown in Fig. 2 . A non-zero χ ″ shows up only on the application of dc magnetic fields. 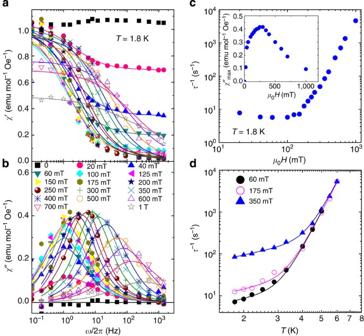Figure 2: Spin–lattice relaxation. (a,b) Realχ’ and imaginaryχ” magnetic susceptibility components of [Co0.05Zn0.95(acac)2(H2O)2] measured atT=1.8 K and under different magnetic fields. Solid lines are least-square Cole–Cole fits18. (c,d) Field and temperature dependences of the spin–lattice relaxation rates obtained from Cole–Cole fits. The inset incshows the field dependence of the maximum imaginary susceptibility component. Solid lines indare least-square fits based on equation (2) with parametersAdir=4.2(1) s−1K−1, 7.2(2) s−1K−1and 47.1(4) s−1K−1for, respectivelyμ0H=60, 175 and 300 mT, andBRaman=5.0(1) × 10−4s−1independent of magnetic field. Figure 2: Spin–lattice relaxation. ( a , b ) Real χ ’ and imaginary χ ” magnetic susceptibility components of [Co 0.05 Zn 0.95 (acac) 2 (H 2 O) 2 ] measured at T =1.8 K and under different magnetic fields. Solid lines are least-square Cole–Cole fits [18] . ( c , d ) Field and temperature dependences of the spin–lattice relaxation rates obtained from Cole–Cole fits. The inset in c shows the field dependence of the maximum imaginary susceptibility component. Solid lines in d are least-square fits based on equation (2) with parameters A dir =4.2(1) s −1 K −1 , 7.2(2) s −1 K −1 and 47.1(4) s −1 K −1 for, respectively μ 0 H =60, 175 and 300 mT, and B Raman =5.0(1) × 10 −4 s −1 independent of magnetic field. Full size image The characteristic spin–lattice relaxation rate τ −1 has been determined by performing Cole–Cole fits [18] of the frequency-dependent susceptibility data. The results are shown also in Fig. 2 . At any magnetic field, τ −1 decreases with decreasing temperature. Below ~400 mK, relaxation becomes sufficiently slow to give rise to a finite magnetization hysteresis ( Fig. 1b ). This dependence can be fitted with the following expression: [11] , [19] where the first and second terms give, respectively, the contributions of one-phonon direct processes, dominant below ~3 K, and of two-phonon Raman processes, which give rise to a strong enhancement of the spin–lattice relaxation above this temperature. In this temperature region, τ −1 versus T data admit also an exponential fit τ −1 ≈ τ 0 −1 exp(− U / k B T ), as expected for a thermally activated Orbach process. However, the activation energies derived from these fits depend on temperature and they amount to ~14–17 cm −1 , thus one order of magnitude smaller than the energy gap between the ground and excited level doublets (see Fig. 1 and Table 1 ). Let us emphasize again the fact that Orbach processes should involve a ‘real’ transition to an intermediate magnetic energy level and that no such level exists at energies below 130 cm −1 from the ground level doublet. The magnetic field dependence of the dynamic susceptibility is remarkable. Despite the fact that τ −1 depends little on magnetic field for μ 0 H ≤100 mT, the relaxation process gives rise to noticeable susceptibility changes only when a magnetic field is applied. The same applies to magnetization hysteresis curves ( Fig. 1b ), whose up and down field-sweeping branches merge as H →0. This behaviour resembles closely that found for some other Co II ions with dominant easy-plane anisotropy [5] , [6] , [7] , [8] , [9] . Two intriguing questions that need to be addressed are, on the one hand, why do Co II spins with D >0 relax so slowly at low T and, on the other, why is this relaxation only visible under finite magnetic fields. In the following, we consider these two questions and propose a mechanism to account for the SMM behaviour of ( 1 ) and of other Kramers ions. Influence of Kramers degeneracy on spin–phonon relaxation Below 30 K, the electronic states of Co II can be described by an effective spin 1/2. The basis states | Ψ › and | Φ › are Kramers-conjugated, that is, | Ψ ›= T | Φ ›, where T is the time-reversal operator [20] . Any spin–phonon operator V sp–ph is invariant under time reversal and therefore it has zero-matrix elements between such states, that is, the selection rule ‹ Ψ | V sp–ph | Φ ›=0 applies [20] . This selection rule, first pointed out by van Vleck [19] in his pioneering work on spin–lattice relaxation [11] (and known ever since as ‘van Vleck cancellation’) implies that the modulation of the crystal field by a phonon cannot induce direct transitions between | Ψ › and | Φ ›. Relaxation between Kramers-conjugate states can nevertheless proceed via Orbach or Raman processes [19] . However, the former are greatly suppressed by the fact that the zero-field splitting is much larger than temperature, and even close to the maximum energies of available phonons (see the inset of Supplementary Fig. 3 ). Only Raman processes retain some finite probabilities on account of their power-law (that is, non-exponential) dependence on temperature. For Kramers ions, they give rise to τ −1 ∝ T [9] (equation (2)) and independent of magnetic field [11] , in good agreement with the experimental behaviour observed above 3–4 K. Yet, experiments (cf Fig. 2 ) show that direct processes are not completely forbidden; instead, they dominate relaxation below 3 K. The origin of this non-perfect cancellation has to be found in the presence of interactions that break time reversal symmetry, thus also the selection rule ‹ Ψ | V sp–ph | Φ ›=0 that follows from it. In the case of Co II , the hyperfine interaction with the I =7/2 nuclear spin turns the electronic doublet into a manifold of 16 electronuclear spin states (see Figs 1d and 3 ). Direct transitions between some of these states are allowed and provide a relaxation channel that remains operative down to absolute zero. The energy splitting associated with the hyperfine interaction enhances also relaxation probabilities between any pair of states because the density of lattice phonons increases with energy [20] . 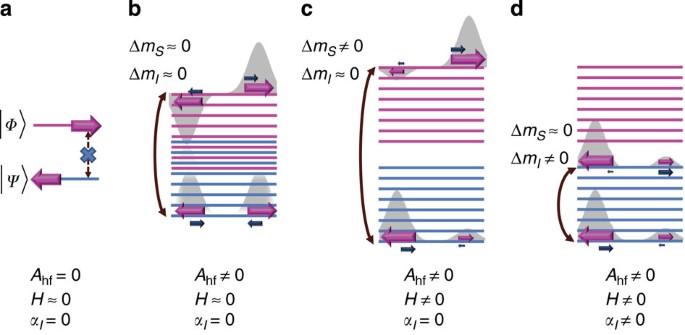Figure 3: Phonon-induced transitions between states of an electronic Kramers doublet. (a) Close to zero magnetic field, electronic states |Ψ› and |Φ› (magenta arrows) are related by time-reversal symmetry. Direct transitions induced by phonons are then forbidden11,19,20. (b) The hyperfine coupling to a nuclear spin (blue arrow) breaks down Kramers degeneracy and allows some phonon-induced transitions between states having approximately the same nuclear spin state (ΔmI≈0). These relaxation paths give rise to vanishingly small magnetic moment changes, because electronuclear spin states are quantum superpositions of |Ψ› and |Φ› (equation (3)). (c) The Zeeman interaction with an external magnetic field further splits the levels, as shown inFig. 1d, and gives each state a net magnetic moment, thus making transitions between them detectable by magnetic susceptibility measurements. At the same time, relaxation rates are enhanced. (d) A non-zero nuclear spin–lattice interaction, characterized by a parameterαI, breaks down the selection rule ΔmI≈0, thus making all transitions allowed. Spin–lattice relaxation is enhanced even further and its initial dependence on magnetic field is reduced. Figure 3: Phonon-induced transitions between states of an electronic Kramers doublet. ( a ) Close to zero magnetic field, electronic states | Ψ › and | Φ › (magenta arrows) are related by time-reversal symmetry. Direct transitions induced by phonons are then forbidden [11] , [19] , [20] . ( b ) The hyperfine coupling to a nuclear spin (blue arrow) breaks down Kramers degeneracy and allows some phonon-induced transitions between states having approximately the same nuclear spin state (Δ m I ≈0). These relaxation paths give rise to vanishingly small magnetic moment changes, because electronuclear spin states are quantum superpositions of | Ψ › and | Φ › (equation (3)). ( c ) The Zeeman interaction with an external magnetic field further splits the levels, as shown in Fig. 1d , and gives each state a net magnetic moment, thus making transitions between them detectable by magnetic susceptibility measurements. At the same time, relaxation rates are enhanced. ( d ) A non-zero nuclear spin–lattice interaction, characterized by a parameter α I , breaks down the selection rule Δ m I ≈0, thus making all transitions allowed. Spin–lattice relaxation is enhanced even further and its initial dependence on magnetic field is reduced. Full size image Electronuclear spin entanglement These simple arguments account for the existence of slow magnetic relaxation in Kramers ions. However, why is such relaxation undetectable at low magnetic fields? A plausible interpretation, sketched in Fig. 3 , reads as follows. Near-zero field, electronuclear states are quantum superpositions of the form where | m I › are nuclear spin states with − I ≤ m I ≤+ I . Contrary to what happens with | Ψ › and | Φ › separately, expectation values for all spin components are very close to zero. The effect is particularly dramatic in the case of easy-plane magnetic anisotropy because states | Ψ › and | Φ ›, which arise from spin projections m S =±½, are very effectively mixed by the hyperfine term of equation (1). Phonon-induced transitions between these states change very little the magnetic susceptibility ( Fig. 3b ). The linear magnetic response is then dominated by reversible, thus independent of frequency, changes of the wave functions induced by the ac magnetic field (van Vleck susceptibility χ VV ). The situation changes as a dc magnetic field is applied. As a result of the Zeeman interaction, electronuclear spin states gradually acquire a non-zero magnetic moment ( Fig. 3c ). First-principles calculations of the spin dynamics This pictorial interpretation is borne out by dynamical susceptibility calculations. The time-dependent populations P n of the electronuclear energy states | Ψ n › have been calculated using a Pauli master equation where the W ’s are transition rates between different states induced by spin–phonon couplings. We use the following spin–phonon Hamiltonian whose particular form is justified in Supplementary Note 3 , where ε αβ and ω αβ (α and β=x, y or z) represent lattice strains and rotations, respectively, and V αβ are spin operators where α I is a parameter that sets the energy scale of nuclear spin–phonon interactions. The first term in equation (6) describes an electron spin–phonon coupling induced by the modulation of the leading magnetic anisotropy term DS z 2 (ref. 21 ). The second term introduces a nuclear spin–phonon interaction. The direct coupling of nuclear spins to phonons is often neglected but, as we argue below, its influence might be crucial to account for the experiments. The transition rates can then be calculated, using first-order time-dependent perturbation theory as described in Supplementary Note 4 , by rewriting ε αβ and ω αβ in terms of creation and annihilation phonon operators and averaging over all relevant phonon modes. We consider three phonon branches with a simple linear phonon dispersion ω = ck and a speed of sound c =1.3 × 10 5 cm s −1 , close to c =2 × 10 5 cm s −1 estimated from the fit of heat capacity data shown in Supplementary Fig. 4 . The rates then read where ρ is the density, ħ ω n ′ n ≡( E n ′ − E n ) is the energy splitting between the final | Ψ n ′ › and initial | Ψ n › electronuclear spin states, f T ( ω n ′ n )=‹ n ( ω n ′ n )› T and ‹ n ( ω nn ′ )› T +1 for ω n ′ n >0 and <0, respectively, and ‹ n ( ω )› T =[exp( ħω / k B T )−1] −1 is the thermal population of phonon modes. The frequency-dependent susceptibility can be derived from the Pauli master equation following a method analogous to that described in ref. 22 , which is detailed in Supplementary Note 5 . The final expression reads where the sum is over all relaxation modes, defined by the solutions of the Pauli master equation, each with a characteristic relaxation time τ ν, Δχ ν is the susceptibility amplitude relaxing at a rate , and χ VV is the van-Vleck susceptibility. Equation (8) provides a suitable basis to discuss how different spin dynamical processes contribute to the ac linear response. The first term is associated with phonon-induced ‘jumps’ between energy levels. The second, χ VV , measures the contribution of quantum processes, including spin tunnelling. Which of the two is slowest depends on the ratio of phonon-induced relaxation rates to Bohr frequencies or, equivalently, of level broadenings γ n ≈ ħ (∑ n ′ W n ′← n ) to energy splittings | ħω n ′ n |. Using the parameters found for complex ( 1 ), we find that γ n <10 −6 cm −1 for all levels from the electronic ground state doublet, thus much smaller than all energy splittings for any magnetic field μ 0 H >10 −3 mT. Under these conditions, which probably apply also to other spin systems with dominant easy-plane anisotropy and fast tunnelling rates, the frequency-dependence of χ ′ and the onset of a nonzero χ ″ are entirely associated with phonon-induced relaxation modes having whereas χ VV is independent of ω and does not contribute to χ ″. The amplitudes of these two contributions, characterized respectively by Δχ ν (or χ ″ max ) and χ VV , measure the fraction of magnetization changes that are either ‘slow’ or ‘fast’. They can strongly depend on the relative magnitudes of those interactions included in the spin Hamiltonian, equation (1). This is illustrated in Fig. 4 . For a Kramers electronic spin ( I =0, Fig. 4a ), χ ″ max > χ VV , because energy states have a net magnetic moment and transitions between them give the dominant contribution to χ . The relaxation rate vanishes as H →0 due to the selection rules associated with time-reversal symmetry, and to the fact that the two lowest lying energy eigenstates are degenerate at zero field (see equation (7)). Introducing the coupling to a I =7/2 nuclear spin ( Fig. 4b ) leads, near-zero field, to entangled electronuclear spin states, with close to zero expectation values for all magnetic moment components. The susceptibility is then dominated by the reversible build-up of a magnetic moment for each of these states, characterized by a large χ VV while phonon-induced transitions (first term in equation (8)) give a smaller contribution. The decrease of χ VV and the increase of χ ″ max with increasing H reflect the onset of a net magnetic moment for each electronuclear state. A situation similar to that found in Fig. 4a is then recovered. In addition, the hyperfine interaction lifts Kramers degeneracy and breaks down the selection rule, thus it enhances τ −1 at low magnetic fields. 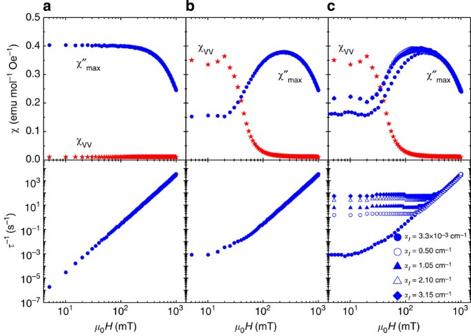Figure 4: Spin dynamics versus hyperfine and nuclear spin-lattice couplings. Field dependence of the reversible van Vleck susceptibilityχVV, the maximumχ” and the average relaxation rateτ−1calculated for different situations: (a)I=0 (electronic spin only); (b)I=7/2 butαI=0 (nuclear spins with no direct coupling to the lattice); (c)I=7/2 and varying values ofαI. The minimumαI=3.3 × 10−3cm−1equals the upper bound of the static quadrupolar interaction constant determined from EPR experiments. Inbandcthe peak (dip) observed inχVV(χ”max) arises from energy level crossings induced by the magnetic field. In all calculations, the magnetic field was oriented at an angleθ=45° andφ=45° with respect to anisotropy axeszandx, respectively, and the speed of sound wasc=1.3 × 105cm s−1. Figure 4: Spin dynamics versus hyperfine and nuclear spin-lattice couplings. Field dependence of the reversible van Vleck susceptibility χ VV , the maximum χ ” and the average relaxation rate τ −1 calculated for different situations: ( a ) I =0 (electronic spin only); ( b ) I =7/2 but α I =0 (nuclear spins with no direct coupling to the lattice); ( c ) I =7/2 and varying values of α I . The minimum α I =3.3 × 10 −3 cm −1 equals the upper bound of the static quadrupolar interaction constant determined from EPR experiments. In b and c the peak (dip) observed in χ VV (χ” max ) arises from energy level crossings induced by the magnetic field. In all calculations, the magnetic field was oriented at an angle θ =45° and φ =45° with respect to anisotropy axes z and x , respectively, and the speed of sound was c =1.3 × 10 5 cm s −1 . Full size image Comparison with experimental results To calculate the average τ −1 and χ ” max of a powder sample, equation (8) was averaged over a random orientation of anisotropy axes and its dependence on frequency fitted with a Cole–Cole law, thus mimicking the experimental procedure. The results, shown in Fig. 5 , confirm that direct relaxation processes contribute at low temperatures. More importantly, they account for the magnetic field dependence of τ −1 and χ ″ max . In particular, they confirm that the increase of χ ″ with H is not associated with a slowing down of magnetic relaxation. Rather, it arises from a gradual evolution of the magnetic response dynamics, marked by the increase of the amplitudes Δχ ν of some relaxation modes at the expense of the reversible contribution χ VV . 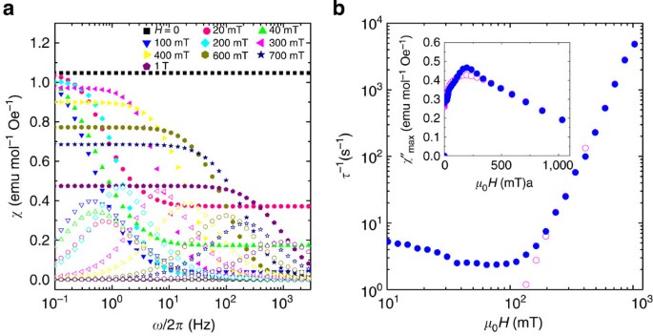Figure 5: First-principles calculations of the spin dynamics. (a) Ac susceptibility of randomly oriented and non-interacting molecules of complex (1) calculated forT=1.8 K and magnetic field strengths varying from 0 up to 1 T. (b) Magnetic field dependence of the spin–lattice relaxation time atT=1.8 K determined from these susceptibility simulations for two values of the nuclear spin–phonon coupling: open symbols,αI=0.05 cm−1; solid symbols,αI=0.5 cm−1. The inset shows the field dependence of the maximum imaginary component for both cases. Figure 5: First-principles calculations of the spin dynamics. ( a ) Ac susceptibility of randomly oriented and non-interacting molecules of complex ( 1 ) calculated for T =1.8 K and magnetic field strengths varying from 0 up to 1 T. ( b ) Magnetic field dependence of the spin–lattice relaxation time at T =1.8 K determined from these susceptibility simulations for two values of the nuclear spin–phonon coupling: open symbols, α I =0.05 cm −1 ; solid symbols, α I =0.5 cm −1 . The inset shows the field dependence of the maximum imaginary component for both cases. Full size image As can be seen in Fig. 4c , the low-field behaviour of τ −1 and, to a lesser extent χ ″ max , turns out to be determined by the strength of the nuclear spin–phonon coupling. We find a reasonable agreement with the experimental results (compare Figs 2 and 5 ) using the coupling given by equation (6) with α I ≈0.5 cm −1 . This coupling is much larger than the maximum energy scales of the quadrupolar ( P ≤3.3 × 10 −3 cm −1 ) and hyperfine ( A ii ≤2.07 × 10 −2 cm −1 ) interactions acting on the nuclear spins in the static case. These results suggest, therefore, the existence of a highly efficient dynamical coupling, a priori unexpected considering the strength of the static quadrupolar interaction, between nuclear spins and molecular vibrations that strongly influences the overall spin relaxation. Its main effect, illustrated in Fig. 3d , is to allow phonon-induced transitions between states differing in their nuclear spin state only, thus breaking the selection rule Δm I =0 that applies when nuclear spins are not coupled to phonons. As the energy differences between such states hardly change with magnetic field (because the nuclear Zeeman effect is very small, see Fig. 1d ), the enhancement of τ −1 introduced by these additional relaxation channels depends little on H . As shown by Fig. 4c and Supplementary Fig. 6 , it dominates until it gets overtaken by the rate of direct transitions between spin-up and spin-down electronic states with Δm I =0. This effect accounts for the nearly constant relaxation rate observed below 100 mT. The slow spin–lattice relaxation of Co II ions with non-uniaxial magnetic anisotropy is the combined result of two main factors. First, the existence of a very strong magnetic anisotropy that, regardless of its sign, gives rise to a Kramers ground level doublet separated from the first excited one by a gap larger than typical acoustic phonon energies. And second, the van Vleck cancellation mechanism, which hinders direct phonon-induced transitions between states of the ground doublet as well as quantum tunnelling processes. Relaxation turns out to be also a remarkable manifestation of electronuclear spin entanglement. Despite its relative weakness, the hyperfine interaction opens paths for magnetic relaxation that would otherwise be forbidden by time reversal symmetry and gives rise to spin states that mask the existence of such relaxation near zero field. Our results reveal also the existence of a rather strong nuclear spin–phonon interaction. Based on the above arguments, it is also possible to suggest possible directions in the search for single-ion spin memories. Besides the two key ingredients mentioned above (half-integer spin and very strong anisotropy), hyperfine interactions need to be minimized to effectively block direct relaxation processes and, at the same time, stabilize states with well-defined spin projections (thus magnetically ‘readable’). Suitable molecular candidates fulfilling such conditions are complexes of Cr III , Ni III and Fe I , which have stable isotopes with zero nuclear spin, and could present a large easy-plane anisotropy for some coordination modes [7] . Recently, Zadrozny et al . [23] have reported a lineal Fe I complex that could satisfy such requirements. Relaxation would then be mainly driven by Raman processes, which can be either ‘frozen’ by lowering temperature or suppressed by linking the molecular memories to substrates with sufficiently high Debye temperatures (thus low densities of thermal phonons). Synthesis All reagents and solvents were purchased from commercial sources and used as received unless otherwise noted. The synthesis of [Co(CH 3 COCHCOCH 3 ) 2 (H 2 O) 2 ] ( 1 ) was performed in a new way not described previously, and the synthesis of the magnetically diluted complex [Zn 1− x Co x (CH 3 COCHCOCH 3 ) 2 (H 2 O) 2 ] ( 2 ) was done following a similar procedure described previously for the synthesis of the Zn complex [24] . The analysis of C, H, N and S were performed with a Perkin-Elmer 24400 series II analyser. Infrared spectra (4,000–400 cm −1 ) of all samples were recorded on a Bruker IFS- 125 FT-IR spectrophotometer. Synthesis of [Co(CH 3 COCHCOCH 3 ) 2 (H 2 O) 2 ] ( 1 ) Cobaltous acetylacetonate (0.5 g, 1.94 mmol) was dissolved in 5 ml of chloroform using an ultrasonic bath, obtaining a pink solution that was left to slow evaporation. After 3–4 days, orange crystals were obtained in a green solution. The solid was filtered out and washed with hexane to yield [Co(CH 3 COCHCOCH 3 ) 2 (H 2 O) 2 ] (270 mg, 0.92 mmol). Anal. calcd (found) for [Co(CH 3 COCHCOCH 3 ) 2 (H 2 O) 2 ]: C, 40.91 (40.95); H, 6.22 (6.19). FT-IR (KBr pellets, cm −1 ): 3,600–3,200, 3,075 w, 2,988 m, 2,924 w, 1,656 m, 1,609 s, 1,520 s, 1,460 s, 1,397 s, 1,261 m, 1,200 m, 1,015 s, 935 s, 770 s, 673w, 658w, 587 m, 564 m, 419 m. Synthesis of [Zn 1− x Co x (CH 3 COCHCOCH 3 ) 2 (H 2 O) 2 ] ( 2 ) NaOH (0.97 g, 24.2 mmol) was dissolved in 20 ml of water and acetylacetone (2.35 g, 23.5 mmol) was added. The solution were stirred 15 min and a solution formed by Zn(NO 3 ) 2 ·6H 2 O (3.31 g, 11.1 mmol) and Co(NO 3 ) 2 ·6H 2 O (0.27 g, 0.93 mmol) in 20 ml of water were added dropwise. A pale pink solid appears immediately. The mixture was stirred during 20 h, filtered out and washed with water, hexane and acetone. X-ray diffraction For compound 1 , a prismatic crystal (0.1 × 0.1 × 0.2 mm 3 ) was selected and mounted on a MAR345 diffractometer with an image plate detector. Unit-cell parameters were determined from 2,959 reflections (3°< θ <31°) and refined by least-squares method. Intensities were collected with graphite monochromatized Mo Kα radiation, using ϕ scan technique. Reflections (5,119) were measured in the range 1.93≤ θ ≤32.06, 1,702 of which were non-equivalent by symmetry (Rint(on I )=0.070 ). Reflections (1,427) were assumed as observed applying the condition I >2 σ ( I ). Lorentz polarization and absorption corrections were made. The structure was solved by Direct methods, using SHELXS computer programme [25] and refined by full-matrix least-squares method with SHELX97 computer programme [26] using 5,119 reflections (very negative intensities were not assumed). The final R (on F ) factor was 0.061, wR (on | F | 2 )=0.203 and the goodness of fit=1.135 for all observed reflections. The number of refined parameters was 87. Maximum shift/esd=0.000, mean shift/esd=0.000. Maximum and minimum peaks in final difference synthesis were 1.486 and −0.668 e Å −3 , respectively, see also Supplementary Table 2 and Supplementary Data 1 . Results for compound 2 are shown in Supplementary Fig. 7 . The powder samples were sandwiched between films of polyester of 3.6 μm of thickness and measured using a PANalytical X’Pert PRO MPD θ/θ powder diffractometer of 240 mm of radius, in a configuration of convergent beam with a focalizing mirror and a transmission geometry with flat samples sandwiched between low absorbing films. Intensities were collected with Cu Kα radiation ( λ =1.5418 Å) and work power of 45 kV–40 mA. Incident beam slits defining a beam height of 0.4 mm. Soller slit 0.02 radians for incident and diffracted beams; PIXcel detector: active length=3.347°; 2 θ/θ scans from 2 to 70°; 2 θ with a step size of 0.026° 2 θ and a measuring time of 200 s per step. A Rietveld refinement was performed using FullProf [27] , see also Supplementary Table 3 . Ab initio calculations A two-step procedure has been carried out to calculate the second-order magnetic anisotropy (or zero-field splitting) parameters ( D and E ). First, we have performed CASSCF/CASPT2 calculations and, second, the energy of these states has been mixed up within the SO-RASSI approach (MOLCAS programme using SINGLE_ANISO code) to introduce the spin–orbit coupling effects. We have employed an all electron ANO-RCC basis set: Co atoms (6 s 5 p 4 d 2 f ), O (4 s 3 p 1 d ), C (3 s 2 p ) and H (2 s ), with an active space considering the seven d electrons of the Co II centres and the 5 d orbitals (7,5). All quadruplets (10) and doublets (40) states have been considered. Experiments Magnetization isotherms were measured using the vibrating sample magnetometer VSM option of the commercial physical property measurement system from Quantum Design. Magnetization and hysteresis studies were extended to the region of very low temperatures 0.4 K< T <10 K using a micro-Hall magnetometer installed in a 3 He refrigerator. Ac and dc susceptibility data were measured with a commercial superconducting quantum interference device magnetometer from Quantum Design (MPMS-XL). The frequency ω /2 π of the ac magnetic field was varied between 0.1 and 1420 Hz, and its amplitude was 2.74 Oe. The diamagnetic contributions of the grease used to prevent sample grains from moving under the action of magnetic field and of the sample holder were characterized in independent measurements. All of them vary linearly with the applied magnetic field and are temperature independent. Their contribution was subtracted from the sample experimental data. EPR data were measured with a Bruker Elexys 580 spectrometer working in X-band. The magnetic field was determined with a Bruker ER035 gaussmeter. It was modulated at 100 kHz with amplitude 0.4 mT. Polycrystalline samples were introduced in a 2-mm diameter quartz tube, which was sealed. An Oxford CF900 continuous flow cryostat refrigerated with liquid Helium was used for cooling the samples. Heat capacity measurements from 203 K down to 0.35 K were performed using the relaxation method of the physical property measurement system platform mentioned above. Accession codes: The X-ray crystallographic coordinates for structures reported in this study have been deposited at the Cambridge Crystallographic Data Centre (CCDC), under deposition number CCDC 1005484. These data can be obtained free of charge from The Cambridge Crystallographic Data Centre via www.ccdc.cam.ac.uk/data_request/cif . How to cite this article: Gómez-Coca, S. et al. Origin of slow magnetic relaxation in Kramers ions with non-uniaxial anisotropy. Nat. Commun. 5:4300 doi: 10.1038/ncomms5300 (2014).